Lipidic cubic phase injector facilitates membrane protein serial femtosecond crystallography Lipidic cubic phase (LCP) crystallization has proven successful for high-resolution structure determination of challenging membrane proteins. Here we present a technique for extruding gel-like LCP with embedded membrane protein microcrystals, providing a continuously renewed source of material for serial femtosecond crystallography. Data collected from sub-10-μm-sized crystals produced with less than 0.5 mg of purified protein yield structural insights regarding cyclopamine binding to the Smoothened receptor. Membrane proteins constitute about one third of the proteome in most organisms, perform critical cellular and physiological functions and represent over 60% of current drug targets in humans [1] . High-resolution three-dimensional structures of membrane proteins are indispensable for understanding their functional mechanisms and designing novel drugs with high selectivity and potency. However, knowledge of membrane protein structures lags behind that of soluble proteins [2] , emphasizing the need to develop innovative methods and approaches. Beginning with the seminal work on photosynthetic reaction centers [3] , membrane proteins have historically been crystallized in detergent micelle solutions. About 17 years ago, an alternative method of crystallization was introduced, based on the use of a membrane-mimetic medium known as the lipidic cubic phase (LCP) [4] , [5] . This technique has proven crucial for determining high-resolution structures and functional mechanisms of membrane proteins from several diverse families, starting with microbial rhodopsins [6] and including G protein-coupled receptors, ion channels, transporters and enzymes [7] , [8] , [9] , [10] , [11] . While LCP crystallization typically produces highly ordered crystals, these crystals are often limited in size. A high density of micrometer-sized crystals in the LCP is often obtained during initial screening, but subsequent optimization to obtain sufficiently large crystals for data collection at synchrotron sources can be laborious and time consuming. Despite the fact that microcrystallography has matured over the last few years [5] , [12] , structure determination of membrane proteins using microcrystals remains difficult. Ultimately, the achievable resolution for well-ordered small crystals is limited by radiation damage [13] that poses an inherent problem for all conventional X-ray-based methods of structure determination. LCP-grown microcrystals are ideally suited for the emerging technique of serial femtosecond crystallography (SFX) [14] , [15] . SFX relies on the fact that the duration of the X-ray pulses generated by an X-ray free-electron laser (XFEL) is so brief (<50 fs), that diffracted photons exit the sample before damage initiated by photoionization can establish itself. Diffraction is thereby recorded from essentially undamaged molecules at or close to room temperature. The peak brightness of an XFEL is a billion times higher than that of third generation synchrotrons, allowing collection of high quality single diffraction patterns from individual sub-10-μm-sized crystals in random orientations. After collecting several hundred thousand of such patterns at a rapid rate, structure factors are determined by Monte Carlo-type integration over the measured diffraction intensities [16] . The first experimental demonstrations of SFX, at low resolution, were carried out with membrane proteins crystallized in detergent solution [17] and in the liquid-like lipidic sponge phase [18] . Recently, the first structures of soluble proteins in aqueous dispersion have been solved at atomic resolution [19] , [20] . To date, the SFX method has been based on X-ray data collection from a liquid stream containing protein micro/nanocrystals. The gas dynamic virtual nozzle (GDVN), which is used to inject microcrystals in their mother liquor into the X-ray beam, produces a liquid jet flowing at 10 m s −1 and focused to 1–5 μm diameter by employing shear and pressure forces from a co-flowing gas [21] . Hence, given the 120 Hz X-ray pulse repetition rate of the Linac Coherent Light Source (LCLS), the sample stream advances several centimeters between X-ray pulses, which are focused to 0.1–2 μm diameter. Consequently, in a typical SFX experiment, only 1 out of 10,000 microcrystals is probed by the X-ray beam. With a liquid flow rate of 10 μl min −1 , it takes 5–6 h to collect a full data set, thus requiring 10–100 mg of pure protein. Obtaining such amounts is not feasible for many membrane proteins. Because of its gel-like nature, LCP allows operation at much lower stream speeds and more efficient sample utilization. Its high viscosity, however, makes it incompatible with GDVN techniques. A new approach was needed to generate a micrometer-sized stream of LCP suitable for SFX. We report here the development of a novel method and a device for extruding LCP at slow flow speeds and with extremely low sample consumption as a continuous 10–50 μm diameter stream. It provides a continuously renewed sample target for interrogation by the femtosecond X-ray beam. The flow speed of the injector is adjustable to the X-ray pulse repetition rate of the XFEL, so that no sample is wasted between shots. LCP-grown microcrystals of the human smoothened (SMO) receptor in complex with cyclopamine have been injected into the femtosecond X-ray beam. Diffraction data from 61,964 microcrystals were merged to recover the structure to 3.2/4.0 Å resolution. The protein consumption is reduced by a factor of 20 compared with SFX experiments with the GDVN nozzle. LCP injection The LCP microextrusion injector ( Fig. 1 ) consists of a hydraulic stage, a sample reservoir and a nozzle. The reservoir can hold up to 20 μl of LCP and is connected to a fused silica capillary with 10–50 μm inner diameter. The LCP is extruded out of this capillary into an evacuated sample chamber and requires a pressure of 2,000–10,000 psi, depending on the nozzle diameter and flow speed. This is provided by the hydraulic stage that amplifies the applied pressure by a factor of 34. Shear force exerted by a co-flowing gas (helium or nitrogen at 300–500 psi supply pressure) keeps the LCP stream on axis (see Methods for details). 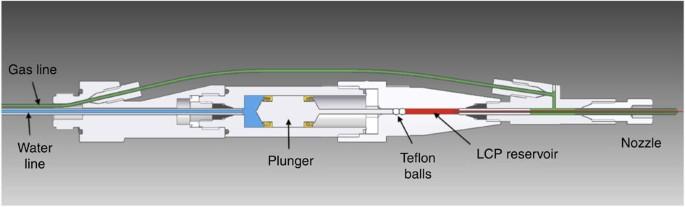Figure 1: Middle section through the LCP injector. In operation, the device is attached via the leftmost threaded fitting to a nozzle rod (not shown) for insertion into the experimental chamber. Water (blue) and gas (green) lines are routed through the nozzle rod from the left. LCP (red) is extruded from the nozzle on the right. Water, at a pressure of up to 300 psi, drives the hydraulic plunger, which amplifies the pressure 34 times to drive LCP through a capillary with an inner diameter of 10–50 μm. Two spherical Teflon beads are used to provide a tight seal against a pressure of up to 10,000 psi. The co-flowing gas is necessary for reliable extrusion and to maintain co-axial flow. Figure 1: Middle section through the LCP injector. In operation, the device is attached via the leftmost threaded fitting to a nozzle rod (not shown) for insertion into the experimental chamber. Water (blue) and gas (green) lines are routed through the nozzle rod from the left. LCP (red) is extruded from the nozzle on the right. Water, at a pressure of up to 300 psi, drives the hydraulic plunger, which amplifies the pressure 34 times to drive LCP through a capillary with an inner diameter of 10–50 μm. Two spherical Teflon beads are used to provide a tight seal against a pressure of up to 10,000 psi. The co-flowing gas is necessary for reliable extrusion and to maintain co-axial flow. Full size image The LCP flow rate (typically 1–300 nl min −1 ) depends on the sample composition, nozzle diameter and pressure and can be optimized for the 120 Hz pulse rate of the LCLS, so that between X-ray pulses, the stream advances only the distance needed to expose fresh sample to the next pulse, dramatically reducing sample consumption compared with GDVN injection ( Supplementary Movie 1 ). The most commonly used lipid for crystallization of membrane proteins in LCP is monoolein, 9.9 MAG (an N.T MAG shorthand notation is used for monounsaturated monoacylglycerol lipids, where ‘N’ is the number of carbon atoms in the acyl chain between the ester and cis -olefinic bonds, and ‘T’ is the number of carbon atoms between the cis -olefinic bond and the end of the chain). However, this lipid is not ideally suited for the LCP–SFX experiments, as it undergoes a phase transition from the cubic phase to a lamellar crystalline (L c ) phase at 18 °C. As LCP is injected into an evacuated sample chamber at ∼ 10 −3 Torr and 20 °C, evaporative cooling can transform it into the L c phase, leading to strong, sharp diffraction rings from the L c phase ( Fig. 2a ). This dramatically increases the background and poses a danger to the detector, which made it necessary to attenuate the LCLS beam by a factor of 20–30. Nonetheless, in our initial experiments both microcrystal samples of β 2 adrenergic receptor (β 2 AR) and adenosine A 2A receptor A 2A AR showed consistent diffraction to ∼ 2.5 Å, even with the highly attenuated beam ( Fig. 2a ). 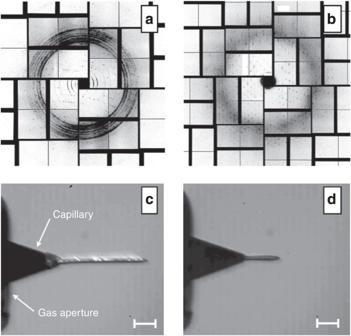Figure 2: Snapshot diffraction patterns and LCP extrusion. (a,b) Single femtosecond snapshot diffraction patterns. (a) Diffraction spots from A2Aadenosine receptor microcrystals in 9.9 MAG/cholesterol LCP to 2.5 Å and strong powder diffraction rings from crystalline lipid. (X-ray intensity attenuated to 7%, 1.5 μm X-ray beam diameter, 50-fs pulse length, 9.5 keV, 15 μm LCP jet diameter, 300 pl min−1flow rate, 1 Hz pulse rate, crystal size: 1 × 1 × 5 μm3). (b) Diffraction from serotonin receptor 5-HT2Bin cholesterol-doped 9.9 MAG+7.9 MAG LCP. No sharp rings are visible suggesting that formation of Lcphase has been avoided (X-ray intensity attenuated to 3.1% due to strong Bragg diffraction from 5 × 5 × 5 μm3sized crystals, 1.5 μm X-ray beam diameter, 50-fs pulse length, 9.5 keV, 50 μm LCP jet diameter, 190 nl min−1flow rate, 120 Hz pulse rate). The resolution at the detector edge in both panels is 2.5 Å. Panels (c) and (d): 9.9 MAG LCP extrusion in vacuum viewed between crossed polarizers. The tapered end of the capillary nozzle is seen protruding out of the gas aperture. Capillary inner diameter: 30 μm. (c) with He as co-flowing gas. Birefringence (bright flecks) is an indication of a transition of the cubic phase to a lamellar crystalline phase due to evaporative cooling. (d) with N2as co-flowing gas and no visible birefringence. Scale bars, 100 μm. Figure 2: Snapshot diffraction patterns and LCP extrusion. ( a , b ) Single femtosecond snapshot diffraction patterns. ( a ) Diffraction spots from A 2A adenosine receptor microcrystals in 9.9 MAG/cholesterol LCP to 2.5 Å and strong powder diffraction rings from crystalline lipid. (X-ray intensity attenuated to 7%, 1.5 μm X-ray beam diameter, 50-fs pulse length, 9.5 keV, 15 μm LCP jet diameter, 300 pl min −1 flow rate, 1 Hz pulse rate, crystal size: 1 × 1 × 5 μm 3 ). ( b ) Diffraction from serotonin receptor 5-HT 2B in cholesterol-doped 9.9 MAG+7.9 MAG LCP. No sharp rings are visible suggesting that formation of L c phase has been avoided (X-ray intensity attenuated to 3.1% due to strong Bragg diffraction from 5 × 5 × 5 μm 3 sized crystals, 1.5 μm X-ray beam diameter, 50-fs pulse length, 9.5 keV, 50 μm LCP jet diameter, 190 nl min −1 flow rate, 120 Hz pulse rate). The resolution at the detector edge in both panels is 2.5 Å. Panels ( c ) and ( d ): 9.9 MAG LCP extrusion in vacuum viewed between crossed polarizers. The tapered end of the capillary nozzle is seen protruding out of the gas aperture. Capillary inner diameter: 30 μm. ( c ) with He as co-flowing gas. Birefringence (bright flecks) is an indication of a transition of the cubic phase to a lamellar crystalline phase due to evaporative cooling. ( d ) with N 2 as co-flowing gas and no visible birefringence. Scale bars, 100 μm. Full size image By changing the co-flowing gas from He to N 2 , the formation of the L c phase was suppressed but not completely eliminated in the case of LCP prepared with 9.9 MAG ( Fig. 2c,d ). However, by replacing the 9.9 MAG with shorter chain MAGs (7.9 MAG [22] or 9.7 MAG (monopalmitolein) available from Avanti Polar Lipids), the formation of the L c phase was completely prevented. Diffraction patterns collected at the LCLS confirmed the presence of the expected cubic-Pn3m phase, without a trace of the L c phase ( Fig. 2b ). In addition, we have established that for crystals that only grow in 9.9 MAG LCP (the most successful crystallization host lipid to date), 7.9 MAG can be added post crystal growth to prevent formation of the L c phase upon injection (see Methods for details), which greatly expands the range of proteins amenable to this method. The high quality of the X-ray diffraction data collected from crystals grown in 9.9 MAG that were delivered in the 7.9/9.9 MAG mixture ( Fig. 2b ) show that the crystals do not suffer from the addition of 7.9 MAG. Diffraction Data and Sample Consumption Using the LCP injector with a flow rate of 170 nl min −1 , SFX data were acquired for several G protein-coupled receptors, including β 2 AR, A 2A AR, SMO, glucagon receptor and serotonin 2B (5-HT 2B ) receptor [23] , as well as the membrane enzyme diacylglycerol kinase (DgkA). Full data sets for SFX structure determination were collected for DgKA, SMO and 5-HT 2B over the course of 5–10 h, while using less than 100 μl of each sample (<0.5 mg of protein). This is a vast improvement over typical sample consumption with a GDVN nozzle, which requires 10 ml (10 mg protein) for a complete data set [17] . A comparison of the amounts of sample used in different experiments with the GDVN and the LCP injector is included in Supplementary Table 1 . As proof of principle for the newly developed LCP–SFX method, we analysed the data collected on human SMO receptor in complex with the naturally occurring teratogen cyclopamine. SMO belongs to the class Frizzled of G protein-coupled receptor superfamily, and participates in embryonic development and tumour growth. The first SMO structure in complex with an antagonist LY2940680 was recently determined by traditional microcrystallography at a synchrotron source [24] . We were, however, unsuccessful in solving the structure of the SMO/cyclopamine complex using synchrotron data collected with a 10 μm diameter X-ray beam due to poor diffraction from relatively large crystals ( ∼ 120 × 10 × 5 μm 3 ; Supplementary Fig. 1c,d ), which presumably suffered from accumulation of crystal growth defects or from effects related to cryocooling. The LCP–SFX data collected on sub-5 μm-sized crystals ( Supplementary Fig. 1a,b ) at room temperature were of a reasonable quality to solve the structure by molecular replacement after application of an anisotropic data truncation at 3.4, 3.2 and 4.0 Å along three principal crystal axes ( Table 1 ). Although the resolution is not very high, it does allow us to confidently locate where this small molecule ligand with an antitumor therapeutic potential [25] binds ( Fig. 3 ). This crystallographic model will be further refined by subsequent biochemical studies. Table 1 Data collection and refinement statistics. 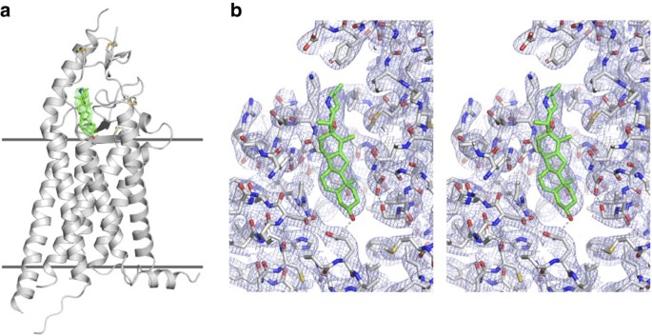Figure 3: Cyclopamine binding to smoothened receptor. (a) Receptor model is shown as a grey cartoon, cyclopamine as a stick model with green carbons, and the ‘omit’ 2mFo–DFcdensity map for cyclopamine contoured at 1σis shown as green wires. Horizontal lines indicate membrane boundaries. (b) Cyclopamine binding pocket is shown in stereo view as a stick model along with 2mFo–DFcdensity map contoured at 1σ.Cyclopamine binds near to the entrance into a long and narrow cavity inside the receptor. Polar interactions stabilizing the shape of the cavity and cyclopamine binding are shown as grey dashed lines. Viewing angles in (a) and (b) are slightly different. Full size table Figure 3: Cyclopamine binding to smoothened receptor. ( a ) Receptor model is shown as a grey cartoon, cyclopamine as a stick model with green carbons, and the ‘omit’ 2mF o –DF c density map for cyclopamine contoured at 1 σ is shown as green wires. Horizontal lines indicate membrane boundaries. ( b ) Cyclopamine binding pocket is shown in stereo view as a stick model along with 2mF o –DF c density map contoured at 1 σ. Cyclopamine binds near to the entrance into a long and narrow cavity inside the receptor. Polar interactions stabilizing the shape of the cavity and cyclopamine binding are shown as grey dashed lines. Viewing angles in ( a ) and ( b ) are slightly different. Full size image In summary, our successful development of an LCP microextrusion injector allows the beneficial attributes of SFX measurements to be coupled with the unique properties and advantages of LCP for membrane protein crystallization. The new technology not only enables the collection of high-resolution structure data from LCP-grown membrane protein microcrystals at room temperature, but also dramatically reduces the amount of protein required, eliminates the need for laborious crystal size optimization and simplifies crystal handling procedures. LCP Injector The LCP injector, consisting of a hydraulic stage, a sample reservoir and a nozzle, is mounted onto the end of the nozzle rod of an injector designed for XFELs [26] . The nozzle rod can be removed from the vacuum chamber without compromising the vacuum, allowing for sample reloading and nozzle change. The hydraulic stage consists of a syringe body with a sealed solid plunger. The syringe body has a large bore on the inlet side and a much smaller bore on the outlet side. The ratio of the respective bore areas gives a nominal amplification factor of 34, delivering 10,200 psi to the LCP reservoir when water on the inlet side is pressurized to 300 psi. The large bore in the syringe body has a diameter of 8 mm. The plunger sliding in this bore has two groves that accept high pressure hydraulic seals (Trelleborg Turcon Variseal) and has a diameter of 8 mm on the water side and an extension with a diameter of 1.37 mm on the LCP side. The plunger extension drives two Teflon beads (Bal-tec) of 1.59 mm outer diameter, which slide in the precision bored 1.37 mm diameter LCP reservoir bore ( Fig. 1 ). The nominal pressure amplification (neglecting frictional forces on the seals) is 34, the ratio of the squared diameters of the bores (8 mm) 2 (1.37 mm) −2 . The Teflon beads seal the bore of the reservoir against LCP leakage. When the beads are pressed into the slightly smaller reservoir bore, they deform cylindrically. The pressure applied by the plunger deforms them further and thus provides a tight seal for pressures up to 10,000 psi on the LCP. The 360 μm outer diameter and 10–50 μm inner diameter fused silica capillary tubing (Polymicro) is kept as short as possible (6 cm) to reduce the pressure necessary to extrude the LCP. The nozzle section and the capillary are connected to the reservoir via standard HPLC conical ports (Upchurch with 10–32 threads). The tapered end of the inner capillary is inserted into a flame-polished square outer glass tube and protrudes out of the exit aperture, so that gas can flow through the open corners at a rate adequate for LCP extrusion (for details of nozzle design, see Weierstall et al . [26] ). The reservoir bore is filled with LCP via a Hamilton syringe and can hold a volume of 20 μl. The Teflon beads are replaced during each sample refill. It is possible to drive the LCP flow in a ‘constant pressure’ mode via pressurized water connected to the plunger inlet. The supply reservoir for the water is, in turn, pressurized by gas from a gas cylinder and the LCP flow rate is controlled by adjusting the gas pressure. However, in this mode of operation the LCP flow rate would occasionally show sudden jumps (possibly due to wall stick-slip [27] of the LCP), leading to sample loss. Better control over LCP flow was achieved in a ‘constant flow rate’ mode implemented by using a HPLC pump (Shimadzu LC-20AD) to drive the hydraulic liquid (water). The LCP flow rate can be optimized for the 120 Hz pulse rate of the LCLS so that between X-ray pulses, the stream advances only the distance needed to expose fresh sample to the next pulse ( Supplementary Movie 1 ). The necessary distance (the ‘damage diameter’) depends on the X-ray beam diameter and pulse energy. Thus, for example, at an X-ray energy of 9.5 keV, a pulse energy of 50 μJ at the sample and a beam diameter of 1.5 μm, this distance is 10–30 μm. Consequently, for a flow speed where the LCP stream travels 10–30 μm between X-ray pulses (1.2–3.6 mm s −1 ), little, if any, sample is wasted and sample consumption is reduced dramatically compared with GDVN injection. Constant LCP flow rates of 1–300 nL min −1 were achieved by adjusting the flow rate setting on the HPLC pump or by using constant pressure mode (for the lowest flow rates). The minimum usable flow rate is set by the diameter of the LCP stream, the distance that the stream must advance between XFEL pulses, and the X-ray pulse repetition rate (for example, for 120 Hz repetition rate, LCP stream diameter of 15 μm and damage diameter of 20 μm, the minimum usable flow rate is 25 nl min −1 ). The LCP flow rate can be calculated by dividing the HPLC pump flow rate by the pressure amplification factor 34. GPCR Expression and Purification Purified GPCR samples (β 2 AR, A 2A AR, glucagon receptor and 5-HT 2B ) [24] , [28] , [29] , [30] , [31] were prepared as follows. Constructs engineered for crystallization were expressed in Sf9 insect cells for 48 h at 27 °C using recombinant baculovirus. Cells were harvested and total membranes were purified by repeated Dounce homogenization and centrifugation in hypotonic and hypertonic buffer. GPCR–ligand complexes were subsequently formed by incubating purified membranes in the presence of ligand, followed by extraction of the complexes in 1% (w/v) N -dodecyl-β- D -maltopyranoside (Anatrace) and 0.2% (w/v) cholesteryl hemisuccinate (CHS, Sigma). Solubilized proteins were purified by immobilized metal affinity chromatography and concentrated to ∼ 20–50 mg ml −1 . GPCR Crystallization Purified protein was reconstituted into LCP by mixing protein solution with molten monoolein (9.9 MAG)/10% (w/w) cholesterol at a volume ratio 2/3 (protein:lipid) using a syringe mixer [32] . Initial crystallization screening was performed using an NT8-LCP robot (Formulatrix) dispensing 40 nl of protein-laden LCP and overlaying it with 800 nl precipitant solution in each well of a 96-well glass sandwich plate (Marienfeld). Plates were stored at 20 °C and periodically imaged in an incubator/imager RockImager 1000 (Formulatrix). Several conditions producing high density of small crystals within 24 h were selected for scaling up ( Supplementary Fig. 1a,b ). Crystals for LCP–SFX were obtained in Hamilton gas-tight syringes by injecting ∼ 5 μl of protein-laden LCP as a continuous column of ∼ 400 μm in diameter into a 100 μl syringe filled with 60 μl of precipitant solution and incubated for at least 24 h at 20 °C. After crystal formation and removal of excess precipitant solution, ∼ 3 μl of molten 7.9 MAG lipid [22] were added to absorb the residual precipitant solution and prevent formation of L c phase upon injection of LCP into vacuum. The resulting crystal containing LCP sample ( ∼ 10 μl) was inspected under visual and ultraviolet microscopes as well as SONICC [33] at the LCLS and loaded in the LCP injector for LCP–SFX data collection. Samples with high crystal density were further diluted two times with LCP prepared from 1:1 ratio of 7.9 MAG and corresponding precipitant solution. Smoothened Receptor An engineered human smoothened receptor construct with truncated amino-terminal cysteine-rich domain (residues 1–189) and carboxy terminus at Q555, and a thermostabilized Escherichia coli apocytochrome B562 (BRIL) [34] fused into intracellular loop 3 (replacing residues from P434 to K440) was generated, expressed and purified as described in the GPCR expression and purification section. The ΔCRD-SMO-BRIL-ΔC construct in complex with cyclopamine readily produced high-density microcrystals in LCP following the crystallization protocol described in the GPCR crystallization section using a variety of precipitant conditions, including 100 mM Hepes pH 7.0, 30% (v/v) PEG 400, 100 mM salt ( Supplementary Fig. 1a,b ). After several rounds of optimization, relatively large crystals obtained in conditions with ammonium salts ( Supplementary Fig. 1c,d ) were used for data collection at a synchrotron source, and microcrystals obtained in 100 mM Hepes pH 7.0, 30% (v/v) PEG 400, 100 mM NaCl were used for LCP–SFX data collection. DgkA Expression and Purification The coding sequence of a thermostable mutant variant of DgkA, with its N-terminal methionine replaced by a hexa-His tag-containing decapeptide (MGHHHHHHEL) to facilitate purification, was synthesized and cloned [10] . This mutant, referred to as Δ7 DgkA, incorporated seven mutations with respect to wild-type DgkA, as follows: A41C, C46A, I53V, I70L, M96L, V107D and C113A. DgkA production and purification, primarily from inclusion bodies, were carried out following published procedures [10] . DgkA Crystallization Crystallization trials began with the reconstitution of the protein into the bi-layer of the lipidic cubic mesophase following a standard protocol [32] . The protein solution at 12 mg ml −1 was homogenized with 7.9 MAG in equal parts by volume using a coupled syringe device at room temperature (20–22 °C). Approximately 20 μl of protein-laden mesophase was transferred into a 0.5 ml Hamilton syringe containing 0.4 ml precipitant solution (0.2% (v/v) MPD, 0.1 M sodium chloride, 0.1 M sodium citrate pH 5.6) using a narrow bore coupler [32] , as described above for GPCR crystallization. The syringe was incubated for 21 days at 20 °C for crystal growth. After separating the bathing solution from the crystal-laden LCP, excess precipitant was absorbed by mixing in 3–5 μl molten 7.9 MAG. This procedure produced optically clear LCP in which microcrystals were dispersed ready for loading into the reservoir of the LCP injector, as described above. Experimental Setup at LCLS and Data Acquisition Rates The experiment took place at the LCLS in the sample chamber of the Coherent X-ray Imaging instrument [35] , using 9.5 keV (1.3 Å) X-ray pulses with a pulse length of 50 fs and repetition rate of 1–120 Hz. The pressure in the experimental chamber was ∼ 10 −5 Torr; the pressure at the extruded LCP sample was about 10 −1 –10 −3 Torr depending on the gas flow rate of the sheath gas. The nozzle area is pumped by a differential pumping system, which reduces gas flow from the nozzle into the main chamber [26] . Due to evaporative cooling, the sample temperature at the point of the X-ray interaction (100 μm downstream of the nozzle exit) is estimated to be slightly below room temperature. An XFEL beam diameter of 1.5 μm was used. With an LCLS frequency of 60–120 Hz (depending on the LCP flow rate), one million diffraction patterns, which is a sufficiently large data set to achieve atomic resolution, can be collected in ∼ 2.5 h with 25 μl of sample. LCP–SFX data for SMO/cyclopamine crystals were collected at an X-ray pulse–repetition rate of 120 Hz. The sample-to-detector distance was 100 mm and the beam was attenuated to 3–6% (2.5–5 10 10 photons per pulse) of the full intensity to avoid detector saturation. A total of 3,510,525 diffraction patterns were collected, of which 274,214 were identified as potential single crystal diffraction patterns with more than 15 potential Bragg peaks by the software Cheetah [36] , corresponding to an average hit rate of 7.8%. Auto indexing and structure factor integration of the crystal hits was performed using CrystFEL (version 0.5.1) [37] , resulting in 61,964 indexed images with a monoclinic lattice (22.6% indexing success rate). Based on the observation of systematic absences ( Supplementary Fig. 2 ) and the behaviour of the Pearson correlation coefficient ( Supplementary Fig. 3 ), we concluded that the diffraction data reach about 3.2 Å resolution, but are highly anisotropic. The UCLA anisotropy server ( http://www.services.mbi.ucla.edu/anisoscale/ ) was used to truncate data at 3.4, 3.2 and 4.0 Å resolution along the three principal axes. Data collection statistics are summarized in Table 1 . Structure determination and refinement The SMO/cyclopamine structure was determined by molecular replacement with the program Phaser [38] using the receptor domain of the previously reported SMO structure in complex with LY2940680 (PDB ID: 4JKV) and the BRIL domain from 5-HT 2B structure (PDB ID: 4IB4) as the search models. After several rounds of alternate refinement by Phenix.refine [39] , including simulated annealing to remove phase bias, and manual inspection and corrections in Coot [40] in the absence of any ligand, extra electron density was observed in the same vicinity of the LY2940680 ligand binding site ( Fig. 3 ). Due to the limited diffraction resolution and a relatively featureless shape of cyclopamine, orienting this ligand in the available elongated density was not straightforward and required combining additional information based on chemical knowledge to create a reasonable model. Since it has been reported that cyclopamine derivatives with bulky substitution groups attached to its secondary amine retain their ability to bind SMO [25] , [41] , cyclopamine was placed in the density with its secondary amine group pointing to the open extracellular space needed to accommodate bulky substitutions. After aligning the major axis of cyclopamine, two alternative orientations of cyclopamine differing by about 180° rotation around its major axis could still be placed in the available electron density. One of these orientations was selected for further refinement based on the favourable conformer energy for cyclopamine, although the second orientation could not be entirely ruled out. The obtained model containing cyclopamine was further refined resulting in R work / R free =0.232/0.278 ( Table 1 ). The structure has an excellent geometry according to the MolProbity server [42] with 95.6% residues in the favored and 4.4% residues in the allowed Ramachandran conformations. Residues 345–354 (intracellular loop 2) and 497–504 (extracellular loop 3) were not modelled due to poor density in these regions. How to cite this article : Weierstall, U. et al . Lipidic cubic phase injector facilitates membrane protein serial femtosecond crystallography. Nat. Commun. 5:3309 doi: 10.1038/ncomms4309 (2014). Accession codes : The coordinates and structure factors of human smoothened receptor in complex with cyclopamine have been deposited in the Protein Data Bank under the accession code 4O9R .